Efimov-driven phase transitions of the unitary Bose gas Initially predicted in nuclear physics, Efimov trimers are bound configurations of three quantum particles that fall apart when any one of them is removed. They open a window into a rich quantum world that has become the focus of intense experimental and theoretical research, as the region of ‘unitary’ interactions, where Efimov trimers form, is now accessible in cold-atom experiments. Here we use a path-integral Monte Carlo algorithm backed up by theoretical arguments to show that unitary bosons undergo a first-order phase transition from a normal gas to a superfluid Efimov liquid, bound by the same effects as Efimov trimers. A triple point separates these two phases and another superfluid phase, the conventional Bose–Einstein condensate, whose coexistence line with the Efimov liquid ends in a critical point. We discuss the prospects of observing the proposed phase transitions in cold-atom systems. A striking analogue to Borremean rings, Efimov trimers are bound configurations of three quantum particles that form near the point of ‘unitary’ interactions [1] , where the pair potential becomes too weak to bind any two of them. Efimov trimers open a window into a largely uncharted world of quantum physics based on many-particle bound states. They were discovered in nuclear physics [2] , [3] , [4] , but have also been discussed in quantum magnets [5] , biophysics of DNA [6] and, most importantly, in ultra-cold atomic gases. In these systems, it has become possible to fine-tune both the sign and the value of the pair interactions through the Feshbach mechanism [7] , from a scattering length a close to zero up to the unitary point | a |= ∞ . In current experiments, Efimov trimers have not been seen directly, but their presence has been traced through the variations of the rate at which the gas loses particles as the interactions are scanned through the unitary region [8] , [9] , [10] , [11] . Theoretical research on Efimov physics has unveiled its universal nature, with the three-particle bound states that form an infinite sequence at unitarity, and that disappear with zero energy at large negative scattering lengths. Beyond the physics of three-bound particles, the ground-state properties of small unitary clusters were studied numerically [12] , and their spectrum computed with a variational ansatz [13] in a trap. However, the macroscopic many-body properties of the unitary Bose gas have remained unknown. The understanding of its thermodynamic behaviour is of great importance, especially as the experimental stability of the unitary Bose gas of cold atoms has been reported for appreciable time scales [11] , [14] , [15] . In this work, we apply a dedicated Path-Integral Monte Carlo algorithm to the unitary Bose gas. This allows us to address the thermodynamics of unitary bosons at finite temperature, both above and below Bose–Einstein condensation. We obtain the phase diagram of a finite number of trapped bosons, and back up our numerical calculations by a general theoretical model that yields a homogeneous phase diagram. At high temperature, we find that the unitary Bose gas is very well described by the available virial coefficients [16] . At lower temperature, the unitary Bose gas undergoes a first-order phase transition to a new superfluid phase, the Efimov liquid, held together by the same effects as Efimov trimers, and whose physical quantities are given by three-body observables. From these two phases, transition lines to a third phase, the conventional Bose–Einstein condensate (BEC), start at a triple point. The coexistence line between the Efimov liquid and the conventional BEC ends in a critical point at high temperature. At a difference with the experimental systems, our model is thermodynamically stable. This is assured through a parameter, the three-body hard core R 0 , that bounds from below the energies of the Efimov states. In cold-atom systems, this parameter is on the order of the van der Waals length l vdW [17] , [18] , [19] . Experimental cold-atom systems are metastable, and particles disappear from the trap into deeply-bound states via the notorious three-body losses. This intricate quantum dynamics, and the description of the losses, are naturally beyond our exact Quantum Monte Carlo approach, and we discuss them on a phenomenological level in order to assess the prospects for experimental tests of our predictions. Model Hamiltonian We describe the system of N interacting bosons by a Hamiltonian where p i , x i and m are the momentum, the position and the mass of particle i , respectively. The pair interaction has zero range and may be viewed, as illustrated in Fig. 1a–c , as a square–well interaction potential whose range r 0 and depth V 0 are simultaneously taken to 0 and ∞ while keeping the scattering length a constant. The unitary point, where the only bound state disappears with zero energy and infinite extension, corresponds to an infinite scattering length a . The three-body interaction V 3 implements a hard-core hyperradial cutoff condition, R ijk > R 0 , where the hyperradius R ijk of particles i , j and k corresponds to their root mean square pair distance . This three-body hard core prevents the so-called Thomas collapse [20] into a many-body state with vanishing extension and infinite negative energy by setting a fundamental trimer energy . The final term in equation (1) models an isotropic harmonic trapping potential of length as it is realized in ultra-cold bosons experiments. The properties of the system described by equation (1) are universal when R 0 is much smaller than all other length scales. 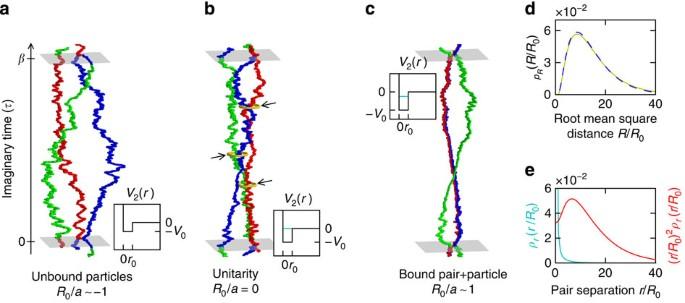Figure 1: Path-integral representation of three bosons at different scattering lengths. The bosons are also atR0/λth=1.3 × 10−2(for the graphical projection of (x,y,zandτ) to three dimensions, see the Methods section). (a) AtR0/a~−1, bosons are unbound and fluctuate on a scaleλth. (b) At unitarity (R0/a=0), pairs of bosons form and break up throughout the imaginary time (yellow highlights, arrows), forming a three-body state bound by pair effects. (c) AtR0/a~1, two bosons bind into a stable dimer (red, blue) and one boson is unbound (green). Insets in (a–c) correspond to finite-range versions of the zero-range interaction used in each case. Cyan levels correspond to the dimer energy. (d) Sample-averaged hyperradial (root mean square pair distance) probabilitypR(R) at constantτ(solid yellow) compared with its analytic zero-temperature value (dashed blue). (e) Sample-averaged pair distributionρr(r), diverging∝1/r2asr→0 and asymptotically constantr-shell probabilityr2ρr(r), in agreement with the Bethe–Peierls condition. Data in this figure concern co-cyclic particles in a shallow trap ofω~0. Figure 1: Path-integral representation of three bosons at different scattering lengths. The bosons are also at R 0 / λ th =1.3 × 10 −2 (for the graphical projection of ( x , y , z and τ ) to three dimensions, see the Methods section). ( a ) At R 0 / a ~−1, bosons are unbound and fluctuate on a scale λ th . ( b ) At unitarity ( R 0 / a =0), pairs of bosons form and break up throughout the imaginary time (yellow highlights, arrows), forming a three-body state bound by pair effects. ( c ) At R 0 / a ~1, two bosons bind into a stable dimer (red, blue) and one boson is unbound (green). Insets in ( a – c ) correspond to finite-range versions of the zero-range interaction used in each case. Cyan levels correspond to the dimer energy. ( d ) Sample-averaged hyperradial (root mean square pair distance) probability p R ( R ) at constant τ (solid yellow) compared with its analytic zero-temperature value (dashed blue). ( e ) Sample-averaged pair distribution ρ r ( r ), diverging ∝ 1/ r 2 as r →0 and asymptotically constant r -shell probability r 2 ρ r ( r ), in agreement with the Bethe–Peierls condition. Data in this figure concern co-cyclic particles in a shallow trap of ω ~0. Full size image Path-integral representation and Efimov trimers In thermal equilibrium, within the path-integral representation of quantum systems that we use for our computations, position variables x i ( τ ) carry an imaginary time index τ ε[0, β =1/ k B T ], where k B is the Boltzmann constant and T is the temperature. The fluctuations of x i (τ) along τ account for the quantum uncertainty. The bosonic nature of many-particle systems manifests itself through the periodic boundary conditions in τ and, in particular, through the permutation structure of particles. The length of permutation cycles correlates with the degree of quantum coherence [21] , [22] , [23] . Interactions set the statistical weights of configurations [24] , [25] . Ensemble averaging, performed by a dedicated Quantum Monte Carlo algorithm, yields the complete thermodynamics of the system (see the Methods section for computational details). The N -body simulation code is massively run on a cluster of independent processors. It succeeds in equilibrating samples with up to a few hundred bosons. Figure 1 presents snapshots of three bosons in a shallow trap at ω ~0 that illustrate the quantum fluctuations in x i (τ), and characterize the Efimov trimer (see the Methods section for a full description of the three bosons simulation). Indeed, for two-body interactions without a bound state, virtually free particles fluctuate on the scale of the de Broglie thermal wavelength that diverges at low temperature (see Fig. 1a ). In contrast, for positive a , a bound state with energy − E dimer =− ħ 2 /( ma 2 ) forms in the two-body interaction potential. Two particles bind into a dimer, and the third particle is free (see Fig. 1c ). At unitarity, the bound state of the pair potential is at resonance E dimer =0, and the scattering length a is infinite (see Fig. 1b ). At this point, the two-body interaction is scale-free. While two isolated particles do not bind in the three-particle system, pairs of particles approach each other and then dissociate, so that, between τ =0 and τ = β , the identity of close-by partners changes several times. This coherent particle-pair scattering process, the hallmark of the Efimov effect [4] , is highlighted in Fig. 1b . At small temperatures, the fluctuations of this bound state remain on a scale proportional to R 0 and do not diverge as λ th . While the two-particle properties are universal at unitarity, the three-boson fundamental trimer state generally depends on the details of the pair interaction. Excited trimers form a geometric sequence of asymptotically universal Efimov trimers with an asymptotic ratio of energies E n / E n +1 ≈515.0 when n → ∞ , where E n is the energy of the n -th excited trimer [1] . Owing to this large ratio, thermal averages cannot identify individual trimer states other than the fundamental trimer at low temperature. For the model Hamiltonian of equation (1), the ground-state trimer is virtually identical to a universal Efimov trimer [12] , and we obtain excellent agreement of the probability distribution of the hyperradius R with its analytically known distribution p R ( R ) (see Fig. 1d ) [1] . This effectively validates our algorithm. Furthermore, the observed quadratic divergence of the pair distance distribution ρ r ( r ), leading to an asymptotically constant r 2 ρ r ( r ) for r →0 (see Fig. 1e ), checks with the Bethe–Peierls condition for the zero-range unitary potential [26] . Equation of state of the unitary Bose gas In local-density approximation, particles experience an effective chemical potential μ ( r )= μ 0 − m ω 2 r 2 /2 that depends on the distance r from the centre of the trap. This allows us to obtain the grand canonical equation of state (pressure P as a function of μ ) from the doubly integrated density profile [27] obtained from a single simulation run at temperature T . We find that the equation of state of the normal gas is described very accurately by the virial expansion up to the third order in the fugacity e βμ (see Fig. 2 and the Methods section) [16] . The third-order term is crucial to the description of Efimov physics as it is the first term at which three-body effects appear [28] . It depends explicitly on T and R 0 . 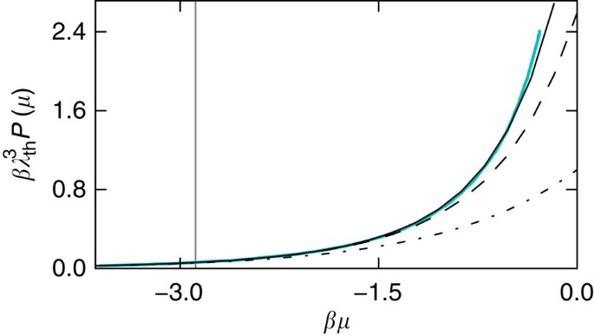Figure 2: Equation of state of unitary bosons in a harmonic trap. The trap is atR0/aωandandN=100. The numerical equation of state of the normal gas forN=100 (solid cyan line) obtained by ensemble averaging of configurations27is compared with the theoretical virial expansion up to the first (dash-dotted black line), second (dashed black line) and third (solid black line) virial coefficients. The vertical grey line indicates the most central region of the trap used to determineμ0by comparison with an ideal gas. Figure 2: Equation of state of unitary bosons in a harmonic trap. The trap is at R 0 / a ω and and N =100. The numerical equation of state of the normal gas for N =100 (solid cyan line) obtained by ensemble averaging of configurations [27] is compared with the theoretical virial expansion up to the first (dash-dotted black line), second (dashed black line) and third (solid black line) virial coefficients. The vertical grey line indicates the most central region of the trap used to determine μ 0 by comparison with an ideal gas. Full size image Phase transitions in the trapped unitary Bose gas In the harmonic trap, particles can be in different thermodynamic phases depending on the distance r from its centre. We monitor the correlation between the pair distances and the position in the trap, and are able to track the creation of a drop of high-density liquid at r ~0 (see Fig. 3a–c ). This drop grows as the temperature decreases. The observed behaviour corresponds to a first-order normal-gas-to-superfluid-liquid transition, and is fundamentally different from the second-order free Bose–Einstein condensation (see Supplementary Fig. 1 ). All particles in the drop are linked through coherent close-by particle switches as in Fig. 1b , showing that the drop is superfluid. Deep inside the liquid phase, the Quantum Monte Carlo simulation drops out of equilibrium on the available simulation times. Nevertheless, at its onset and for all values of R 0 , the peak of the pair correlation function is located around 10 R 0 , which indicates that the liquid phase is of constant density (see Fig. 3c ). At larger values of R 0 , the density difference between the trap centre and the outside vanishes continuously, and the phase transition is no longer seen (see Fig. 3d–f ). Beyond this critical point, the peak of the pair correlation also stabilizes around 10 R 0 , which indicates a cross-over to liquid behaviour (see Fig. 3f and the Methods section for additional details on the characterization of the first-order phase transition). 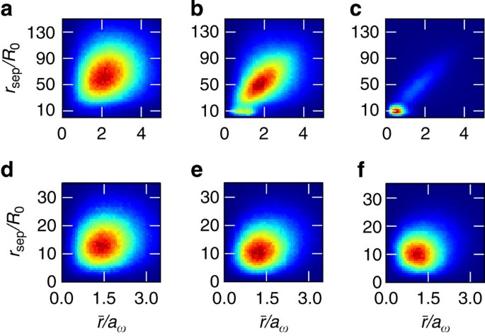Figure 3: Two-dimensional histogram of pair distances and centre-of-mass positions forN=100 bosons. The pair distance is given byrsepand the centre-of-mass position is given by. Upper panels: first-order phase transition forR0/aω=0.07. (a) At, the distribution is that of the normal phase. (b) At a slightly lower temperature, a second peak with smaller pair distances ~10R0appears in the trap centre. (c) At, most particles are in the trap centre, with small pair distances ~10R0. Lower panels: smooth dependence of pair distances and densities on temperature. AtR0/aω=0.23, the pair distances decrease smoothly between(d) and(e) and has stabilized around 10R0at(f). Figure 3: Two-dimensional histogram of pair distances and centre-of-mass positions for N =100 bosons. The pair distance is given by r sep and the centre-of-mass position is given by . Upper panels: first-order phase transition for R 0 / a ω =0.07. ( a ) At , the distribution is that of the normal phase. ( b ) At a slightly lower temperature , a second peak with smaller pair distances ~10 R 0 appears in the trap centre. ( c ) At , most particles are in the trap centre, with small pair distances ~10 R 0 . Lower panels: smooth dependence of pair distances and densities on temperature. At R 0 / a ω =0.23, the pair distances decrease smoothly between ( d ) and ( e ) and has stabilized around 10 R 0 at ( f ). Full size image Model for the normal-gas-to-Efimov-liquid transition Our numerical findings suggest a theoretical model for the competition between the unitary gas in third-order virial expansion and an incompressible liquid of density and constant energy per particle − ε ∝ E t , as suggested by ground-state computations for small clusters [12] (see Supplementary Fig. 2 ). For simplicity, we neglect the entropic contributions to the liquid-state free energy ε ≫ TS , so that F 1 ≈− N ε . The phase equilibrium is due to the difference in free energy and in specific volume at the saturated vapour pressure (see the Methods section and Supplementary Fig. 3 ). We extend the third-order virial expansion to describe the gaseous phase in the region where quantum correlations become important. Because the conventional Bose–Einstein condensation is continuous, it still conveys qualitative information about the transition into the superfluid Efimov liquid in that region. At small R 0 →0, the coexistence line approaches infinite temperatures as the fundamental trimer energy diverges. For larger values of R 0 , the density of the liquid decreases and approaches the one of the gas. The liquid–gas transition line ends in a critical point, where both densities coincide. As the liquid is bound by quantum coherence intrinsic to the Efimov effect, this critical point must always be inside a superfluid, that is, between the Efimov liquid and the BEC, which become indistinguishable. The agreement between this approximate theory and numerical calculations for the trap centre phase diagram is remarkable (see Fig. 4a ). Beyond the critical point, we no longer observe a steep drop in the density on decreasing the temperature. We also notice that quantum coherence builds up in the gaseous phase, so that only a conventional Bose–Einstein condensation takes place. Our numerical results suggest it occurs at a temperature slightly lower than that for the ideal Bose gas [29] , . 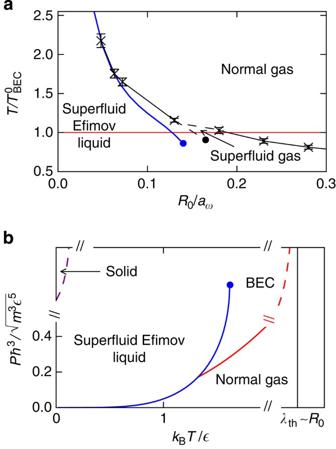Figure 4: Phase diagram of unitary bosons in the trap centre and in homogeneous space. (a) In the harmonic trap, depending on the value ofR0/aω, we observe a normal-gas-to-superfluid-liquid first-order phase transition or a conventional second-order Bose–Einstein phase transition (solid black lines). The error bars indicate the last value ofTat which the system was a pure normal gas, and the first value ofTat which we observed either the superfluid Efimov liquid or the BEC. The normal-gas-to-superfluid-liquid phase transition corresponds well to our theoretical model (solid blue line) at high temperatures. Consistently with theoretical predictions, the numerical coexistence lines are qualitatively continued to a triple point and a critical point (dashed black lines). (b) In a homogeneous system, the normal-gas-to-superfluid-liquid coexistence line (solid blue) and the conventional Bose–Einstein condensation line (solid red) are universal. The predicted divergence of the normal-gas-to-superfluid-liquid coexistence line (dashed red) and the phase transition to a solid phase (dashed purple) are non-universal physics specific to our interaction model. Figure 4: Phase diagram of unitary bosons in the trap centre and in homogeneous space. ( a ) In the harmonic trap, depending on the value of R 0 / a ω , we observe a normal-gas-to-superfluid-liquid first-order phase transition or a conventional second-order Bose–Einstein phase transition (solid black lines). The error bars indicate the last value of T at which the system was a pure normal gas, and the first value of T at which we observed either the superfluid Efimov liquid or the BEC. The normal-gas-to-superfluid-liquid phase transition corresponds well to our theoretical model (solid blue line) at high temperatures. Consistently with theoretical predictions, the numerical coexistence lines are qualitatively continued to a triple point and a critical point (dashed black lines). ( b ) In a homogeneous system, the normal-gas-to-superfluid-liquid coexistence line (solid blue) and the conventional Bose–Einstein condensation line (solid red) are universal. The predicted divergence of the normal-gas-to-superfluid-liquid coexistence line (dashed red) and the phase transition to a solid phase (dashed purple) are non-universal physics specific to our interaction model. Full size image Homogeneous phase diagram of the unitary Bose gas Our theoretical model also yields a phase diagram for a homogeneous system of unitary bosons (see Fig. 4b ) where, in addition, the conventional Bose–Einstein condensation is simply modelled by that of free bosons [30] . In absence of a harmonic trap, only two independent dimensionless numbers may be built, k B T / ε , and . As a consequence, the phase diagram in these two dimensionless numbers is independent of the choice of ε , that is, of R 0 . The scaling of the dimensionless pressure with and of the dimensionless temperature with explains that the triple point appears much farther from the critical point in the homogeneous phase diagram than in the trap. We expect model-dependent non-universal effects in two regions. At high temperature λ th << R 0 , only a classical gas should exist as the quantum fluctuations are too small to build up quantum coherence and, in particular, permutations between particles. At high pressure P ∝ T , we expect a classical solid phase driven by entropic effects, as for conventional hard-sphere melting. To situate the theoretical results presented in this work in an experimental context, we present the data of Fig. 4b in terms of R 0 n 1/3 and λ th n 1/3 (see Fig. 5 ). In this diagram, systems with identical values of T and R 0 and different densities correspond to straight lines passing through the origin. In the unstable region, we expect a homogeneous system described by the Hamiltonian of equation (1) to phase-separate on the same such line into the superfluid Efimov liquid and the normal gas or the BEC. 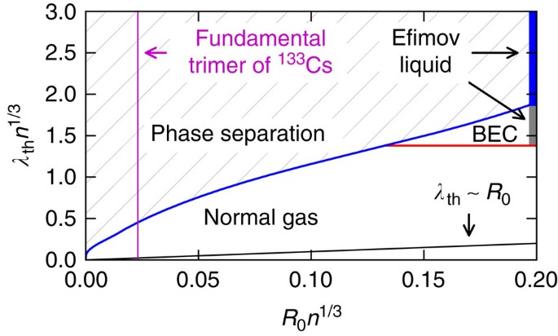Figure 5: Homogeneous phase diagram of unitary bosons: comparison with experimental densities. Data ofFig. 4bexpressed through the dimensionless numbersλthn1/3andR0n1/3. In the coexistence region, the system phase separates into the superfluid Efimov liquid (thick blue line) and, depending on temperature, the normal gas or the BEC. At high density, the BEC undergoes a cross-over to Efimov liquid behaviour (thick grey line). The value ofR0n1/3~0.023 corresponding to the fundamental trimer of133Cs at densityn=1013cm−3is indicated by the vertical magenta line. Figure 5: Homogeneous phase diagram of unitary bosons: comparison with experimental densities. Data of Fig. 4b expressed through the dimensionless numbers λ th n 1/3 and R 0 n 1/3 . In the coexistence region, the system phase separates into the superfluid Efimov liquid (thick blue line) and, depending on temperature, the normal gas or the BEC. At high density, the BEC undergoes a cross-over to Efimov liquid behaviour (thick grey line). The value of R 0 n 1/3 ~0.023 corresponding to the fundamental trimer of 133 Cs at density n =10 13 cm −3 is indicated by the vertical magenta line. Full size image In cold-atom systems, the atomic interactions have deeply-bound states not present in our model, and the strict hyperradial cutoff is absent. Nevertheless, an effective three-body barrier at a universal value ~2 l vdW [18] induces a universal relation between the fundamental trimer energy E t and the van der Waals length l dvW [17] , [19] , [31] , [32] . In Fig. 5 , a vertical line marks the experimentally realistic value R 0 n 1/3 ~0.023 obtained for 133 Cs atoms at a density n =10 13 cm −3 , using R 0 ~2 l vdW and l vdW =101 a 0 [7] , where a 0 is the Bohr radius. Other atomic species yield smaller values of R 0 n 1/3 , for which this discussion is also valid. An experimental system may be quenched along this line into the unstable region by suddenly increasing the scattering length up to unitarity via the Feshbach mechanism. If this quench starts from a weakly interacting BEC at very low temperature, the four-body recombination process (that saturates at a rate ) will dominate the three-body recombination process (that saturates at a rate ) [11] , [33] , [34] , [35] , a condition that may be written as nK 4 ≳ K 3 (cf. refs 36 , 37 ). Whereas the latter is responsible for the three-body losses into deeply-bound dimer states, the former may represent one possible strategy for creating Efimov trimers. In the unstable region, the recombination process would create liquid droplets of ever increasing size. Deep inside the unstable region, far away from the coexistence line, we expect this growth to be a fast, barrier-free, runaway process involving spinodal decomposition [38] , [39] , rather than a slow activation process of nucleation over a free-energy barrier produced by the competition of bulk and surface energies. In a thermodynamically stable system, complete separation on macroscopic length scales proceeds through a coarsening process on length scales that slowly increase with time [38] , [40] . At the Bose–Einstein condensation temperature of the non-interacting gas, this would lead to a large liquid fraction 1− n g / n , where n g is the density of the gas at coexistence, and n the density of the system before phase separation. However, this will certainly not be observable in current cold-atom experiments, as sufficiently large droplets of dense liquid are unstable towards decay into deeply-bound atomic states. Nevertheless, the instability of the gas and the creation of microscopic liquid droplets might be quite realistic. These could be observed as they would lead to an important increase of the three-body losses, proportional to in the liquid phase. The time scales for the creation of a minority liquid phase after a quench is a classic problem of non-equilibrium statistical mechanics. In the present context, it is rendered even richer by the fact that the initial low-temperature phase is a weakly interacting superfluid, and that even the normal gas phase is thermodynamically unstable. These questions are closely related to the very existence of the unitary Bose gas on time scales larger than its thermalization time. Very recent experimental works indicate that the ultra-cold unitary Bose gas can indeed be stabilized on appreciable time scales [11] , [14] , [15] . Path-integral Monte Carlo algorithm In our path-integral quantum Monte Carlo simulation, the contribution of the three-body hard-core interaction to the statistical weights of discretized path configurations are computed using Trotter’s approximation, which consists in simply rejecting configurations with R < R 0 . The contribution of the zero-range unitary interaction is computed using the pair-product approximation, which estimates the weight of two nearby particles without taking other particles into consideration. Both approximations are valid when the discretization step is small [23] . In the simulation, new configurations are built from existing configurations according to several possible update moves. A new one, the compression-dilation move, was introduced to specifically address the divergence of the pair correlation function at small distances (see Fig. 1e ; Supplementary Fig. 4 ). For each set of parameters, the simulation was run on up to 16 independent processors for up to 10 days to reduce the statistical error. Simulation of three bosons In our simulations of unitary bosons, the system is contained in a harmonic trap. This regulates the available configuration space. For the same purpose, in the three-body calculations at ω ~0 presented in Fig. 1 , we impose that the three bosons are on a single permutation cycle: in Fig. 1a–c the blue, red and green bosons are, respectively, exchanged with the red, green and blue bosons at imaginary time β . This condition does not modify the properties of the fundamental trimers at unitarity, as other permutations could be sampled at no cost at points of close encounter such as those highlighted in Fig. 1b . Figure 1a–c presents four-dimensional co-cyclic path-integral configurations in three-dimensional plots. In this graphic representation, the centre of mass, whose motion is decoupled from the effect of the interactions, is set to zero at all τ . The three spatial dimensions are then reduced to two dimensions by rotating the triangle formed by the three particles at each imaginary time to the same plane in a way that does not favour any of the three spatial dimensions while conserving the permutation cycle structure and the pair distances. High-temperature equation of state Within the local-density approximation, the grand canonical equation of state P ( μ ) may be obtained from the numerical doubly integrated density profile [27] as where μ ( x )= μ 0 − m ω 2 x 2 /2 is the local chemical potential along direction x , and μ 0 the chemical potential at the centre of the trap, measured from a fit of the equation of state to that of an ideal gas in the outer region of the trap. We compare this numerical equation of state to the cluster expansion that expresses the pressure in terms of the fugacity e βμ (see Fig. 2 ): The l -th cluster integral b l follows from the virial coefficients of smaller order. It represents l -body effects that cannot be reduced to smaller non-interacting groups of interacting particles [28] . We use the analytical expressions of b 2 and b 3 at unitarity that have become available [16] . Monitoring the phase transitions When the densities of the gas and the superfluid Efimov liquid approach each other, observing directly the two-dimensional histogram of pair distances and centre-of-mass positions does not allow to distinguish between a weakly first-order phase transition and a cross-over (see Supplementary Fig. 5 ). In this regime, we monitor the normal-gas-to-superfluid-liquid phase transition more accurately by following the evolution of the first peak of the pair correlation function (obtained by ensemble averaging) with temperature (see Supplementary Fig. 6 ). In Fig. 4 , Bose–Einstein condensation is assumed when particles lie on a permutation cycle of length >10 with probability 0.05 (ref. 22 ). Analytical model for the transition into the Efimov liquid First-order phase transitions take place when the free energy F of a homogeneous physical system is not a convex function of its volume V . Splitting the system into two phases is then favourable over keeping it homogeneous (see Supplementary Fig. 3 ). In this situation, at coexistence and in absence of interface energy, the chemical potentials and the pressures of both phases are equal. The virial expansion is an excellent approximation to describe the normal gas phase of unitary bosons far from the superfluid transition. Although this expansion becomes irrelevent in the superfluid gas, its analytic continuation conveys important qualitative features because of the continuous nature of conventional Bose–Einstein condensation, and is therefore a suitable approximation for the conventional BEC. The theoretical model for the superfluid liquid is that of an incompressible liquid of specific volume ν 1 and negligible entropic contribution to the free energy F 1 =− N ε . Simulations yield , and the negligible contribution of the entropy to the free energy is ensured for non-pathological systems at low temperature. The results in ref. 12 may be extrapolated to ε =10.1 E t (see Supplementary Fig. 2 ), a value adjusted to ε =8 E t in Fig. 4a to account for finite-size effects. In practice, we draw the transition line into the superfluid liquid by finding the smallest chemical potential at which the presssures of the incompressible liquid and of the normal gas coincide at a temperature T : As n =1/ ν = ∂ μ P , the crossing to the regime where this equation has no solution corresponds to the critical point, where both densities are equal. To draw the coexistence line for the trap centre with N =100 particles in Fig. 4a , its chemical potential μ 0 is found from integrating the density throughout the trap: where the local chemical potential μ ( r )= μ 0 − m ω 2 r 2 /2 is computed within the local density approximation. How to cite this article: Piatecki, S. and Krauth, W. Efimov-driven phase transitions of the unitary Bose gas. Nat. Commun. 5:3503 doi: 10.1038/ncomms4503 (2014).